Evidence for a nematic component to the hidden-order parameter in URu2Si2from differential elastoresistance measurements For materials that harbour a continuous phase transition, the susceptibility of the material to various fields can be used to understand the nature of the fluctuating order and hence the nature of the ordered state. Here we use anisotropic biaxial strain to probe the nematic susceptibility of URu 2 Si 2 , a heavy fermion material for which the nature of the low temperature ‘hidden order’ state has defied comprehensive understanding for over 30 years. Our measurements reveal that the fluctuating order has a nematic component, confirming reports of twofold anisotropy in the broken symmetry state and strongly constraining theoretical models of the hidden-order phase. The heavy fermion compound URu 2 Si 2 undergoes a continuous phase transition at T HO ~17 K, the precise nature of which has not been fully established, despite considerable experimental [1] , [2] , [3] , [4] and theoretical [5] , [6] , [7] , [8] , [9] , [10] , [11] , [12] attention. Determination of the symmetry (or symmetries) that are broken in the ‘hidden order’ phase is not just of purely academic interest, but also has a direct bearing on the symmetry of the superconducting gap that develops below T c =1.5 K. Of particular relevance to the present work, several recent measurements have provided evidence that the hidden-order phase breaks the fourfold rotational symmetry of the high-temperature tetragonal crystal lattice [13] , [14] , [15] , [16] ; however, the degree of anisotropy that is observed depends heavily on the crystal size (as determined via torque measurements [13] ) and also on the crystal quality (for X-ray diffraction measurements [14] ), leading to some contention as to whether or not these are intrinsic effects. In the current work, we take a complementary approach and probe the fluctuating order in the temperature regime above T HO . Our results demonstrate first that the fluctuating order has a nematic component, confirming that the hidden-order phase spontaneously breaks fourfold rotational symmetry, and second that other symmetries must also be broken at the phase transition. To measure a general susceptibility of a system, one must apply the appropriate conjugate field (that is, the physical quantity that couples linearly to the given order) and measure the linear response. For a tetragonal material, such as URu 2 Si 2 above the hidden-order transition, the conjugate field to electronic nematic order is anisotropic biaxial in-plane strain (either ε aniso =( ε xx − ε yy ) or ε aniso = γ xy for spontaneous order in the [100] or [110] directions, corresponding to B 1 g and B 2 g representations of the D 4 h point group, respectively). The nematic susceptibility for each of these orientations is then , where represents any thermodynamic quantity measuring the induced anisotropy in mutually orthogonal directions ([100] and [010], or [110] and , respectively [17] ; also see ‘Elastoresistance Measurements’ subsection in the Supplementary Discussion ). For a continuous electronic nematic phase transition, χ N diverges towards the phase transition, signalling an instability towards nematic order. Such behaviour was recently observed for the representative underdoped iron pnictide Ba(Fe 1− x Co x ) 2 As 2 , demonstrating that the structural phase transition that precedes the onset of collinear antiferromagnetic order in that material is driven by electronic nematic order [17] , [18] , [19] . There are also classes of order for which there is a single transition to an ordered state that has a nematic component, while simultaneously breaking additional symmetries. A simple example would be a unidirectional incommensurate density wave with order parameter Δ i =Δ( Q i ), for which both translational and tetragonal symmetries are simultaneously broken at the same transition ( Q i corresponds to the ordering wave vector of the density wave, and i = x or y ). In such a case, anisotropic strain is not conjugate to the order parameter (that is, the coupling term in the free-energy expansion is not bilinear). Nevertheless, the inherent nematicity associated with the unidirectional density wave motivates introduction of a nematic order parameter , which couples linearly to (|Δ x | 2 −|Δ y | 2 ) and to which anisotropic strain is linearly coupled (see ‘Nematic × (?) Symmetry’ subsection in the Supplementary Discussion ). For such a situation, and with the assumption of a continuous transition, an analysis based on standard Ginzburg–Landau theory for coupled order parameters reveals that the nematic susceptibility follows a Curie–Weiss temperature dependence at high temperatures (as the density wave fluctuations orient in the anisotropic strain field), but then develops an additional divergence close to the transition temperature, experimentally distinguishing the behaviour from that of a ‘pure’ nematic transition. We find that hidden order in URu 2 Si 2 appears to fall into this latter class, having a nematic component but also breaking additional symmetries at the hidden-order phase transition (see ‘Nematic Susceptibility: Theory’ subsection in the Supplementary Discussion ). Our measurements are based on a novel technique that probes the differential response in the electrical resistivity to anisotropic biaxial strain in mutually perpendicular directions. We measure the induced resistivity anisotropy, , which, by symmetry, is proportional to in the limit of asymptotically small values. The induced anisotropy is characterized by specific terms in the associated elastoresistivity tensor m ij that relate changes in the resistivity to strains experienced by the material [19] . In the regime of infinitesimal strains (linear response), the elastoresistivity coefficients ( m 11 − m 12 ) and 2 m 66 are linearly proportional to the bare (unrenormalized) nematic susceptibility, and , for strains in the [100] and [110] directions, respectively [19] . The proportionality constant relating the resistivity anisotropy to the nematic order parameter is governed by microscopic physics, but does not contain any singular contributions. Consequently, any divergence of the induced resistivity anisotropy is directly related to divergence of the nematic susceptibility. Since this is ultimately a derivative of a transport measurement, the technique is especially sensitive to static or fluctuating order that affects the Fermi surface. As we describe in this study, our measurements reveal a strongly anisotropic differential elastoresistance between the B 1 g and B 2 g symmetry channels. In the B 2 g channel for temperatures well above T HO , the 2 m 66 elastoresistivity coefficient follows a Curie–Weiss dependence. This behaviour directly implies that the fluctuating order has a nematic component. However, we also find a striking additional divergence in 2 m 66 close to the phase transition, which tracks the heat capacity. This additional contribution to the differential elastoresistance demonstrates that while hidden order in URu 2 Si 2 must break fourfold rotational symmetry, it also breaks other symmetries and hence is not purely nematic. Representative measurements of (Δ R / R ) yy for five different temperatures are shown in Fig. 1b,c for and [100] oriented crystals, respectively, revealing a linear response. The sign of (Δ R / R ) xx is opposite to that of (Δ R / R ) yy due to the anisotropic strain (that is, the imposed symmetry breaking), distinct from changes in resistance observed under conditions of hydrostatic pressure [20] . This procedure was performed for both the (Δ R / R ) xx and (Δ R / R ) yy orientations on the same sample by removing the crystal from the piezo with acetone between each measurement. The slopes Δ R / R versus strain for each orientation were found using a linear fit and the difference was taken. The resulting elastoresistivity coefficients 2 m 66 and m 11 − m 12 are plotted in Fig. 2 as a function of temperature. 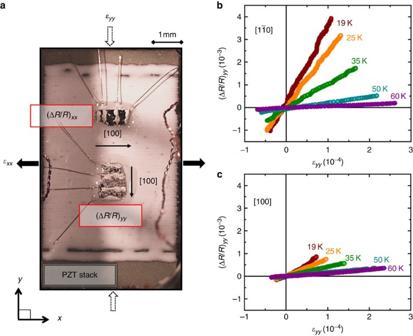Figure 1: Measurement of elastoresistivity coefficients. Anisotropic strain is achieved by gluing thin crystals of URu2Si2to the side of a PZT piezoelectric stack such thatεxxis opposite in sign toεyy. The Cartesian axes are defined relative to the piezo stack itself, with thex-(y-)direction parallel to the short (long) axis of the piezo. (a) Photograph of [100] oriented URu2Si2crystals mounted in the (ΔR/R)yyand (ΔR/R)xxdirections on the surface of a PZT piezoelectric stack. Strain gauges mounted on the opposite face of the piezo stack measureεyyandεxx, which are related by the effective Poisson ratio of the PZT stack,νp≡−εxx/εyy. (b) and (c) show representative (ΔR/R)yyelastoresistance data for five different temperatures as a function ofεyyforand [100] orientations, respectively. Data are plotted for both warming and cooling cycles and are identical within the resolution of the experiment. The resistive response to anisotropic strain is considerably larger (by a factor of ~4) for measurements made in thedirection compared with the [100] direction. Figure 1: Measurement of elastoresistivity coefficients. Anisotropic strain is achieved by gluing thin crystals of URu 2 Si 2 to the side of a PZT piezoelectric stack such that ε xx is opposite in sign to ε yy . The Cartesian axes are defined relative to the piezo stack itself, with the x -( y -)direction parallel to the short (long) axis of the piezo. ( a ) Photograph of [100] oriented URu 2 Si 2 crystals mounted in the (Δ R / R ) yy and (Δ R / R ) xx directions on the surface of a PZT piezoelectric stack. Strain gauges mounted on the opposite face of the piezo stack measure ε yy and ε xx , which are related by the effective Poisson ratio of the PZT stack, ν p ≡− ε xx / ε yy . ( b ) and ( c ) show representative (Δ R / R ) yy elastoresistance data for five different temperatures as a function of ε yy for and [100] orientations, respectively. Data are plotted for both warming and cooling cycles and are identical within the resolution of the experiment. The resistive response to anisotropic strain is considerably larger (by a factor of ~4) for measurements made in the direction compared with the [100] direction. 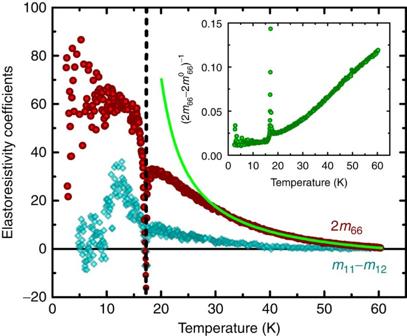Figure 2: Temperature dependence of the elastoresistivity coefficients. The 2m66(red circles) and them11−m12(cyan diamonds) elastoresistivity coefficients reveal a large directional anisotropy, with 2m66reaching very large values close to and below the hidden-order transition. The dashed vertical black line indicates the hidden-order transition,THO=17.17 K, determined from the peak in the temperature derivative of the resistivity. The green curve is a fit of 2m66to a Curie–Weiss temperature dependencefrom 60 to 30 K, as described in the main text. The fit is extrapolated below 30 K to emphasize deviations from Curie–Weiss behaviour below this temperature. The best-fit values for the parameters areC=375 K,θ=15.2 K and. The inset showsversus temperature, withdetermined from the green fit in the main figure. Full size image Figure 2: Temperature dependence of the elastoresistivity coefficients. The 2 m 66 (red circles) and the m 11 − m 12 (cyan diamonds) elastoresistivity coefficients reveal a large directional anisotropy, with 2 m 66 reaching very large values close to and below the hidden-order transition. The dashed vertical black line indicates the hidden-order transition, T HO =17.17 K, determined from the peak in the temperature derivative of the resistivity. The green curve is a fit of 2 m 66 to a Curie–Weiss temperature dependence from 60 to 30 K, as described in the main text. The fit is extrapolated below 30 K to emphasize deviations from Curie–Weiss behaviour below this temperature. The best-fit values for the parameters are C =375 K, θ =15.2 K and . The inset shows versus temperature, with determined from the green fit in the main figure. Full size image The data shown in Figs 1 and 2 reveal a striking anisotropy in the elastoresistivity coefficients, with 2 m 66 values considerably larger, and also more strongly temperature dependent, than m 11 − m 12 . For comparison, the elastoresistivity coefficients of simple metals are small (of order one) and essentially isotropic [19] . It is worth remarking that the differential elastoresistance of URu 2 Si 2 is comparable to that of BaFe 2 As 2 , for which the response along the [100] and [110] orientations is also strongly anisotropic, with 2 m 66 values reaching ~40 approaching the tetragonal-to-orthorhombic phase transition in that material. Recalling that 2 m 66 is proportional to the nematic susceptibility in the [110] direction , the large values of 2 m 66 (red data points in Fig. 2 ) and the strong temperature dependence both indicate a diverging nematic susceptibility in the B 2 g ( d xy symmetry) channel, and hence motivate fitting the data to the Curie–Weiss form . Since the elastoresistance only develops significant values below ~60 K, the range of temperatures over which this fit can be applied is necessarily small. Nevertheless, if we attempt fits over different temperature ranges, the best fit, defined by a reduced χ 2 statistic closest to 1, occurs for a range from ~30 K to the maximum of 60 K, with a Weiss temperature θ =15.2±0.3 K (see ‘Curve Fitting’ subsection in the Supplementary Discussion ). Extrapolation of the best fit function to lower temperatures (shown as a green line in Fig. 2 ) reveals significant deviation from Curie–Weiss-like behaviour for temperatures below ~30 K. The onset of this deviation at 30 K is coincident with a suppression in ( T 1 T ) −1 seen in recent NMR experiments [21] , suggestive of a common origin, possibly associated with the progressive development of strongly fluctuating order. In contrast, m 11 − m 12 , which is proportional to , is small and exhibits only a weak temperature dependence (cyan data points in Fig. 2 ); additional measurements on a separate crystal confirmed the small value of m 11 − m 12 (see ‘Elastoresistance Measurements’ subsection in the Supplementary Discussion ). Given the large values of 2 m 66 , it is likely that this weak temperature dependence derives from slight sample misalignment (that is, a small amount of contamination from 2 m 66 in the [100] orientation due to imperfectly constrained current paths within the crystal). For the remaining discussion we focus solely on the 2 m 66 data. The most striking aspect of the temperature dependence of the elastoresistivity coefficients is the sharp downward anomaly observed at T HO . The 2 m 66 data are replotted in Fig. 3a on an expanded scale for the temperature window from 15.5 to 19 K, spanning T HO . The anomaly exactly aligns with the sharp peak in the temperature derivative of the in-plane resistivity d ρ /d T ( Fig. 3b,c ), indicating that the effect is associated with the thermodynamic phase transition at T HO . For comparison, heat-capacity measurements were also performed for the same crystal that was used for the oriented measurements. The data closely follow the temperature dependence of d ρ /d T (ref. 22 ), reminiscent of the theoretical treatment of critical fluctuations in metallic antiferromagnets by Fisher and Langer [23] , with slight differences in the peak position attributed to small differences in thermometry between the two different systems used for transport and thermodynamic measurements. 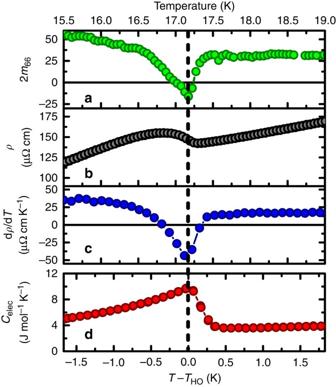Figure 3: Temperature dependence of 2m66and heat capacity nearTHO. Temperature dependence of (a) the 2m66elastoresistivity coefficient, (b) the in-plane resistivityρ, (c) the temperature derivative of the in-plane resistivity dρ/dTand (d) the electronic specific heat in the immediate vicinity ofTHO, all measured on the sameoriented crystal. The phonon component to the specific heat was subtracted out by using ThRu2Si2, such thatCelec(URu2Si2)=(C(URu2Si2)−C(ThRu2Si2)). Data for all four panels are plotted as a function ofT−THO, with the absolute temperature scale for the transport measurements shown on the upper axis. The temperature range in absolute units for all four plots is the same. The position (THO=17.17 K) and width of the peak in 2m66exactly match that of dρ/dT, while there is a slight temperature offset (THO=17.47 K) relative to the heat capacity measurement (but with the same width). Differences betweenTHOobtained from transport and electronic specific heat are attributed to slight differences in thermometry between the two measurements. Figure 3: Temperature dependence of 2 m 66 and heat capacity near T HO . Temperature dependence of ( a ) the 2 m 66 elastoresistivity coefficient, ( b ) the in-plane resistivity ρ , ( c ) the temperature derivative of the in-plane resistivity d ρ /d T and ( d ) the electronic specific heat in the immediate vicinity of T HO , all measured on the same oriented crystal. The phonon component to the specific heat was subtracted out by using ThRu 2 Si 2 , such that C elec (URu 2 Si 2 )=( C (URu 2 Si 2 )− C (ThRu 2 Si 2 )). Data for all four panels are plotted as a function of T − T HO , with the absolute temperature scale for the transport measurements shown on the upper axis. The temperature range in absolute units for all four plots is the same. The position ( T HO =17.17 K) and width of the peak in 2 m 66 exactly match that of d ρ /d T , while there is a slight temperature offset ( T HO =17.47 K) relative to the heat capacity measurement (but with the same width). Differences between T HO obtained from transport and electronic specific heat are attributed to slight differences in thermometry between the two measurements. Full size image The observation of the Curie–Weiss temperature dependence of the 2 m 66 elastoresistivity coefficient, combined with the large anisotropy between 2 m 66 and m 11 − m 12 , strongly implies a nematic character to the fluctuations associated with the hidden-order phase. However, the sharp downward anomaly in 2 m 66 at T HO , which apparently closely follows the anomaly in the heat capacity at T HO , is not consistent with a ‘pure’ nematic behaviour, implying that hidden order does not couple bilinearly to anisotropic strain. Motivated by these results, we consider below a Ginzburg–Landau model of a more complex system described by a multicomponent (vector) order parameter (see ‘Nematic × (?) Symmetry’ subsection in the Supplementary Discussion ). As described previously, the nematic susceptibility of a material that suffers an electronic nematic instability follows a Curie–Weiss temperature dependence, as has been observed for the iron pnictides [17] , [18] , [19] . However, a nematic response is also possible if the ordered state breaks fourfold spatial rotation symmetry, but does not couple to strain as a bilinear term in the free energy. In this scenario, the hidden order state would be described by a two-component vector-order parameter . Motivated by the inherent nematicity in such a system, the nematic response can be modelled in mean field theory by introducing a separate nematic order parameter , which couples to the strain in the form where λ is a coupling constant. The theory does not depend on the microscopic origin of , which could be an independent-order parameter or parasitic to the hidden order. Within such a theory, an additional contribution to the nematic susceptibility occurs close to the hidden-order transition, which is proportional to the singular part of the heat capacity (Δ C V ) associated with the critical behaviour: where the constant β depends on the strengths of the couplings between , , and ε aniso (see ‘Nematic × (?) Symmetry: Functional Form’ subsection in the Supplementary Discussion ). This effect is analogous to anomalies observed in the elastic moduli and thermal expansion coefficients at a structural phase transition, first described by Testardi [24] . Intuitively, the relationship between the nematic susceptibility and heat capacity arises because it is the square of hidden order that generates a nematic distortion; within mean field considerations, both nematic and energy density fluctuations (that is, the heat capacity) are related to the square of the order parameter (see ‘Nematic × (?) Symmetry: Mean Field Intuition’ subsection in the Supplementary Discussion ), so these two quantities necessarily mirror each other near the phase transition. The close correspondence between the predictions of this Ginzburg–Landau treatment and the observed data strongly suggest that hidden order in URu 2 Si 2 is described by a two-component order parameter that breaks fourfold symmetry. Since the 2 m 66 coefficient diverges but m 11 − m 12 does not, the orientation of the nematic fluctuations is along the [110] and directions, consistent with the orientation deduced by measurements in the broken symmetry state [13] . The significance of this result is not so much the deduction that other symmetries are broken in the hidden-order phase. Over a period of many years, a growing body of evidence points to partial gapping of the Fermi surface and a possible doubling of the unit cell in the c -direction [3] , [25] , [26] , [27] , [28] , [29] , [30] , [31] , [32] , [33] , [34] , [35] , [36] . Rather, our result is significant because it confirms the more controversial conclusions drawn from earlier torque [13] , NMR [15] , cyclotron resonance [16] and X-ray diffraction [14] measurements that the hidden-order phase spontaneously breaks fourfold lattice symmetry. Our results, which are ultimately based on statements about symmetry, do not identify a specific microscopic model for hidden order, but they clearly place tight constraints, namely that the hidden-order phase is described by a vector-order parameter that breaks fourfold symmetry. The same coupling to the crystal lattice that yields the resistive response to strain must also cause an orthorhombic distortion below T HO , consistent with reports of high-resolution X-ray diffraction measurements [14] . Whether or not this anisotropy is observed in thermodynamic measurements of macroscopic crystals is then a matter of the resolution of the specific measurement and the relative population of the two orthogonal orthorhombic domain orientations (which will be influenced by both crystal size and quality, via effects associated with pinning of domain walls). Both aspects illustrate the distinct advantage of probing the nematic susceptibility in the temperature regime T > T HO , for which there are no domains (one is simply probing the susceptibility of the symmetric phase) and for which the resistivity anisotropy is extremely sensitive to subtle perturbations of the Fermi surface. Despite these advances, important questions remain. In particular, since nematic fluctuations in the B 2 g channel couple linearly to the shear modulus, one anticipates a softening of the C 66 elastic constant approaching the hidden-order phase transition. However, earlier measurements of the elastic moduli [37] , [38] do not show such a softening. At least in principle, weak coupling between the nematic-order parameter and the crystal lattice (consistent with the small magnitude of the orthorhombic distortion observed in X-ray diffraction experiments [14] ) would limit any appreciable renormalization of C 66 to small values of the reduced temperature close to the phase transition (see ‘Nematic Susceptibility: Theory’ subsection in the Supplementary Discussion ). Nevertheless, the present results, in conjunction with other measurements that reveal a twofold anisotropy in the hidden-order phase [13] , clearly motivate a careful reinvestigation of the elastic properties of URu 2 Si 2 for samples of a comparably high RRR. To probe a thermodynamic susceptibility, one measures the response of an order parameter to an application of its conjugate field. In this context, the elastoresistivity measurements presented here track the induced resistivity anisotropy as a function of anisotropic biaxial strain. For a tetragonal material, the elastoresistivity tensor (which relates the normalized resistivity change to the strain experienced by a material) is defined by Anisotropic strain is achieved by gluing thin crystals of URu 2 Si 2 to the surface of a PZT piezoelectric stack. The high-quality crystals used for these experiments were characterized by residual resistance ratios (RRR) of 170 (for the oriented measurements) and 81–87 (for the [100] oriented measurements; see Supplementary Table I ). The elastoresistivity coefficients m 11 − m 12 and 2 m 66 are determined from the difference of (Δ R / R ) yy and (Δ R / R ) xx for a given set of strains for [100] and oriented crystals, respectively [19] . To first order this is also equal to the induced resistivity anisotropy N , expressed below in terms of the anisotropic biaxial strain ( ε yy − ε xx ): where x and y refer to the axes along which the piezo stack induces biaxial strain, indicated in Fig. 1a and following the description given in previous work [19] . For each temperature, five voltage cycles were performed. Voltage applied to the piezo stack was increased/decreased in a stepwise manner. The time delay between steps was varied from 0.25 to 2 s with no change in the measured elastoresistance, indicating the absence of any appreciable heating effects. Data shown in all figures were taken using a delay of 0.5 s. The strain was measured using mutually perpendicular strain gauges glued to the back surface of the piezo stack. How to cite this article: Riggs, S. C. et al . Evidence for nematic component to the hidden-order parameter in URu 2 Si 2 from differential elastoresistance measurements. Nat. Commun. 6:6425 doi: 10.1038/ncomms7425 (2015).